Phylogenetic constraints on ecosystem functioning There is consensus that biodiversity losses will result in declining ecosystem functioning if species have different functional traits. Phylogenetic diversity has recently been suggested as a predictor of ecosystem functioning because it could approximate the functional complementarity among species. Here we describe an experiment that takes advantage of the rapid evolutionary response of bacteria to disentangle the role of phylogenetic and species diversity. We impose a strong selection regime on marine bacterial lineages and assemble the ancestral and evolved lines in microcosms of varying lineage and phylogenetic diversity. We find that the relationship between phylogenetic diversity and productivity is strong for the ancestral lineages but brakes down for the evolved lineages. Our results not only emphasize the potential of using phylogeny to evaluate ecosystem functioning, but also they warn against using phylogenetics as a proxy for functional diversity without good information on species evolutionary history. In the face of extremely elevated extinction rates worldwide there is an urgent need to understand the relationship between diversity and ecosystem functioning (EF). There is today a consensus that biodiversity losses will result in declining EF if species perform different roles in ecosystems, in other words if they have different functional traits [1] , [2] , [3] . Understanding the mechanisms that shape the distribution of species traits within species assemblages has thus become central to the biodiversity–EF research agenda. Although ecological studies have traditionally looked at how species assemble into communities and impact EF, evolutionary studies have concentrated on the diversification processes responsible for the range of functional traits we observe in nature [4] , [5] . The emerging fields of evolutionary community ecology and ecophylogenetics integrate these distinct perspectives of biodiversity to provide tools for its conservation and the provision of ecosystem services [4] , [5] , [6] , [7] , [8] , [9] . Until now, different approaches have been used to understand the role of evolutionary history on EF. Experimental adaptive radiations in microbial metacommunities and mesocosm experiments with fishes have shown that increases in EF occur in tandem with the emergence of niche complementarity [10] , [11] . Palkovacs et al . [12] have also shown that coevolution between two stream fishes could strongly impact the relative effect of invasion on stream ecosystem processes. Given the opportunity for experimental evolution in a laboratory setting, bacteria have also been used to show how diversification into specialist and generalist strategies, consequently alter the shape of the diversity–productivity relationship [13] . An alternative approach has been to evaluate, a posteriori , the contribution of evolutionary history (phylogenetic diversity, PD) of artificially assembled communities to EF. It is hypothesized that if closely related species are ecologically similar (that is, trait conservatism), EF such as productivity should increase with PD [14] . As we usually have imperfect knowledge of the distribution of functional traits responsible for resource acquisition and species interactions, the knowledge of the evolutionary relationships could thus be used as a proxy for functional diversity [4] , [9] , [14] . Accordingly, comparative analyses have shown that phylogenetic relatedness was a reasonable proxy of functional trait diversity and therefore a good predictor of EF [14] , [15] , [16] . In fact, even when measures of functional diversity are available, PD can outperform functional diversity in predicting EF [17] . This approach is important as PD could then serve as an integrative measure to help conservation of particular ecosystem properties [18] , [19] , [20] , [21] . Although these new approaches have opened very important research avenues they come with inherent limitations. The experimental studies that have demonstrated that past environmental conditions could affect species' contribution to EF lack explicit consideration of the community evolutionary history. On the other hand, functional and species diversity tend to be correlated in experimental biodiversity–EF experiments, making it difficult to distinguish their relative contribution to EF with the a posteriori approach. Here, we describe an experiment that took advantage of the rapid evolutionary response of bacteria to disentangle the role of phylogenetic and species diversity by directly manipulating the evolutionary history (that is, the degree of trait conservatism) among species. We performed a biodiversity–EF experiment with a set of marine bacterial lineages that were evolved under selective conditions [13] . Sixteen bacterial lineages were isolated from coastal seawater and their ribosomal small subunit genes were sequenced to construct a phylogenetic tree. The bacteria used in the study are environmental isolates with closest small subunit matches to the genera Pseudoalteromonas (3 strains) and Psychrobacter (13 strains). Both genera are commonly found among the cultivable fraction of copiotrophic bacteria from natural environments (fast growing aerobic heterotrophs), ranging from marine waters to clinical systems. We imposed a selection regime by growing each lineage on a different, randomly assigned carbon source for 64 days. We then conducted assays for each strain on the different carbon sources over 48 h (a few generations). The main response to selection was that strains became more specialized on particular substrates. We finally conducted biodiversity functioning experiments for the ancestral and evolved linages, with lineage diversity as a categorical treatment (2, 4 and 8 lineages) and PD as a continuous variable. Phylogenetic to productivity relationship Our experimental design allowed us to investigate the independent effects of lineage and PD for both the ancestral and the evolved lineages. We found for the ancestral lineages that productivity increased significantly with lineage diversity ( Fig. 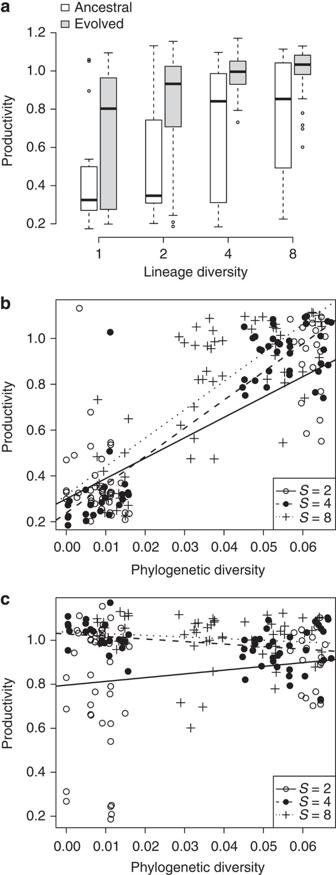Figure 1: Relationship between diversity and productivity. (a) Relationship between productivity and lineage diversity for both the ancestral and the evolved lineages. Productivity is approximated by measuring light absorbance at 660 nm after 48 h of incubation in marine broth media. Note that monocultures are added to the figure for the purpose of comparison but absent from the statistical analysis because they have null phylogenetic diversity. (b) Productivity increases with phylogenetic diversity for the ancestral lineages with species richnessS=2, 4 and 8 lineages (R2=0.71 for the ANCOVA model, seeTable 1), but not for (c) experimentally evolved lineages (Table 1). The fitted lines represent the linear models per lineage diversity treatment. 1a ; Table 1 ) and PD ( Fig. 1b ; Table 1 ). The PD explained much more variance in productivity than lineage diversity (F 1,189 =412.54 and F 3,189 =7.42, respectively). There was a significant interaction between phylogenetic and lineage diversity, indicating the slope of the PD–EF relationship increased with lineage diversity ( Table 1 ). The productivity also increased significantly with diversity of evolved lineages ( Fig. 1a ), but, in contrast to the ancestors, we found no effect of PD on productivity ( Fig. 1c ; Table 1 ). There was a weak but significant (at P =0.05) interaction between lineage diversity and PD ( Table 1 ). The PD–EF was only significantly different from 0 for the four lineages treatment (a negative slope). Figure 1: Relationship between diversity and productivity. ( a ) Relationship between productivity and lineage diversity for both the ancestral and the evolved lineages. Productivity is approximated by measuring light absorbance at 660 nm after 48 h of incubation in marine broth media. Note that monocultures are added to the figure for the purpose of comparison but absent from the statistical analysis because they have null phylogenetic diversity. ( b ) Productivity increases with phylogenetic diversity for the ancestral lineages with species richness S =2, 4 and 8 lineages ( R 2 =0.71 for the ANCOVA model, see Table 1 ), but not for ( c ) experimentally evolved lineages ( Table 1 ). The fitted lines represent the linear models per lineage diversity treatment. Full size image Table 1 Summary of the ANCOVA models. Full size table Transgressive overyielding A positive relationship between diversity and EF can be explained by both complementarity and sampling (or positive selection) effects [2] . The signature of complementarity is usually investigated through the pattern of overyielding in the mixtures (ref. 22 ; see Methods). Transgressive overyielding occurs when the productivity in mixture is larger than the maximal productivity of the constituent species. We found that transgressive overyielding (positive values of the overyielding index) rarely occurred for both ancestral and evolved lineages ( Fig. 2 ). Note that our analysis assumes the most productive lineage excludes all others by competition, as it does not account for the relative abundance of the lineages at the end of the experiment, and consequently is not a true measurement of the sampling effect [22] . There was almost no overyielding for all mixtures (a majority of assemblages had a negative overyielding index). There was no significant effect of lineage diversity on the overyielding index for both ancestral and evolved lineages ( Table 1 ; Fig. 2a ). The relationship between PD and the overyielding index was significant for the ancestral but not for the evolved lineages ( Table 1 ; Fig. 2b,c ). There was, however, a highly significant interaction between lineage diversity and PD for the ancestral lineages. Only high ancestral lineage diversity treatments (4 and 8 lineages) had a positive relationship between PD and the overyielding index ( Fig. 2b ). We analyzed the robustness of this result by running the analysis of covariance (ANCOVA) analysis for only the assemblages that did not contain the highly productive clade (lineages 30, 77 and 94) and found that the PD no longer had an effect on productivity (F 1,72 =0.72; P =0.40). This result strongly suggests that a sampling effect is the most important driver of the PD–productivity relationship we found. 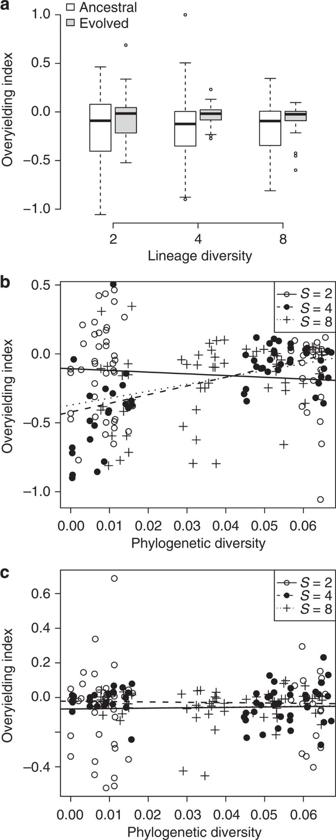Figure 2: Relationship between diversity and transgressive overyielding. (a) Relationship between the overyielding index and lineage diversity for both ancestral and evolved lineages. There is no significant relationship between phylogenetic diversity and productivity for (b) the ancestral lineages with species richnessS=2, 4 and 8 lineages (R2=0.14 for the ANCOVA model, seeTable 1) and (c) experimentally evolved lineages (R2=0.02). Positive values indicate transgressive overyielding. The fitted lines represent the linear models per lineage diversity treatment. Figure 2: Relationship between diversity and transgressive overyielding. ( a ) Relationship between the overyielding index and lineage diversity for both ancestral and evolved lineages. There is no significant relationship between phylogenetic diversity and productivity for ( b ) the ancestral lineages with species richness S =2, 4 and 8 lineages ( R 2 =0.14 for the ANCOVA model, see Table 1 ) and ( c ) experimentally evolved lineages ( R 2 =0.02). Positive values indicate transgressive overyielding. The fitted lines represent the linear models per lineage diversity treatment. Full size image Sampling versus complementarity effects The absence of overyielding suggests that a sampling effect is driving the positive relationship between diversity and productivity. This would imply a 'phylogenetic sampling effect', meaning higher average productivity at high PD because of increased likelihood of having the productive lineage in the mixture. We indeed found that the distribution of productivity in monoculture of ancestral lineages was conserved in the phylogeny ( Fig. 3 ; Mantel test between phylogenetic distance and difference of productivity in monoculture, r-Mantel=0.93, P =0.003). The most productive ancestral lineages were part of an isolated clade (lineages 30, 77 and 94), suggesting that the PD–EF relationship was dominated by a selection effect. The probability of having one of these highly productive lineages was higher at elevated PD for the ancestral lineages. There are several hypotheses to explain this result, for instance, some carbon substrates on the Ecoplates might be closer to the dominant ones found in the marine broth (MB) media, or simply favoured a stronger selection response. As the selection regime was independent of the phylogeny (each lineage was randomly assigned to a single-carbon substrate), it randomized the metabolic profiles of the lineages within the phylogeny and consequently their performance on the MB media. 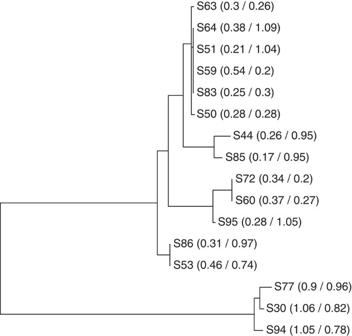Figure 3: Phylogeny of the 16 lineages used in this study. Productivity in monoculture (numbers between parentheses, for ancestral/evolved lineages) indicates there is a clade of ancestral lineages with conserved high productivity. This pattern is lost with experimental evolution. Figure 3: Phylogeny of the 16 lineages used in this study. Productivity in monoculture (numbers between parentheses, for ancestral/evolved lineages) indicates there is a clade of ancestral lineages with conserved high productivity. This pattern is lost with experimental evolution. Full size image We also tested if, in addition to conservatism of maximal productivity, there is also conservatism for other traits. We therefore performed individual assays on 31 carbon substrates to quantify the functional complementarity among strains [13] . We found a significant relationship between the similarity in substrate usage and phylogenetic distance for the ancestral lineages (r-Mantel=−0.510, P =0.018). This functional conservatism was partly due to the fact that the strains 30 and 94 shared similar carbon usages ( Figs 4 and 5 ). The diversity of carbon substrate usages was increased by the selection treatment. The trait conservatism was however lost for the evolved lineages ( Figs 3 and 5 ; for productivity: r-Mantel=−0.09, P =0.898; for carbon usage: r-Mantel=−0.1539, P =0.068). These results are consistent with the experimental design of the selection treatment as the assignment of carbon substrates to the different lineages was performed randomly with respect to the phylogeny. They suggest that the conservatism of productivity in monocultures is not only the main driver of a 'phylogenetic sampling effect' for the ancestral strains ( Fig. 1b ), but also that trait complementarity explains the residual relationship between PD and productivity ( Fig. 2b ). 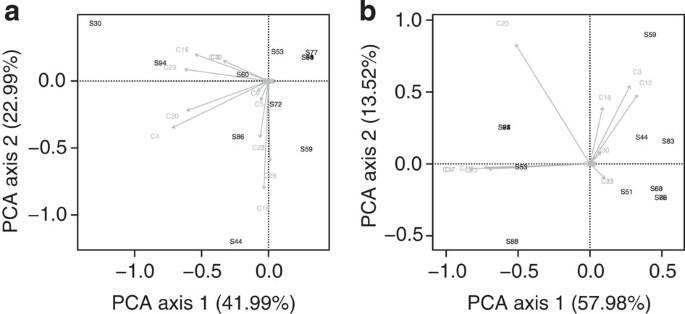Figure 4: PCA illustrating the functional complementarity among lineages. The PCA is performed on the carbon substrates usage by the (a) ancestral and (b) evolved lineages. Note that only the substrates that were used by at least one lineage are represented. PCA, principal component analysis. Figure 4: PCA illustrating the functional complementarity among lineages. The PCA is performed on the carbon substrates usage by the ( a ) ancestral and ( b ) evolved lineages. Note that only the substrates that were used by at least one lineage are represented. PCA, principal component analysis. 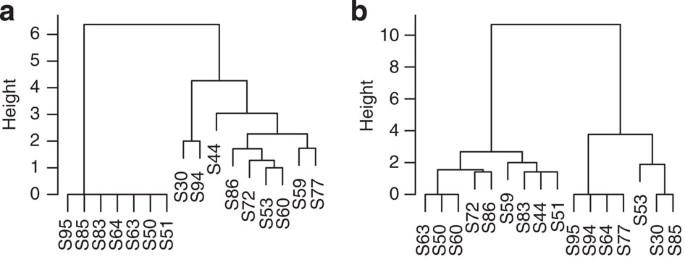Figure 5: Hierarchical clustering of the carbon substrates usage. Clustering of the carbon substrates usage is shown by the (a) ancestral and (b) evolved lineages. The clustering was computed using the Ward algorithm on Euclidean distance matrices of binary data of carbon usage. Note there is no significant relationship between the dendrograms (both) and the phylogenetic tree (r-Mantel test). Full size image Figure 5: Hierarchical clustering of the carbon substrates usage. Clustering of the carbon substrates usage is shown by the ( a ) ancestral and ( b ) evolved lineages. The clustering was computed using the Ward algorithm on Euclidean distance matrices of binary data of carbon usage. Note there is no significant relationship between the dendrograms (both) and the phylogenetic tree (r-Mantel test). Full size image Here, we took advantage of rapid evolutionary response of bacteria to disentangle experimentally the role of phylogenetic relatedness and species richness on EF. This research provides a first and robust experimental test of the positive relationship between PD and EF in the face of divergent selection pressures. Our results demonstrate that there are evolutionary conditions where PD ceases to be closely associated with EF. Experimental evolution on different resources resulted in the distribution of traits across the phylogeny being essentially randomized, leading to the loss of the relationship between PD and EF. The empirical PD–EF relationship observed in the ancestral lineages was therefore not robust when lineages experienced directional selection in different environments. Previous studies have implicitly assumed that either PD will be a useful tool for predicting EF, or else we will have to resort to identifying and measuring functional traits [17] . Although our results emphasize the importance of PD to predict EF, they also set the limits for this approach. We suspect that our experiment represents the two ends of a continuum where the importance of phylogenetic to explain EF varies. In communities where there is an evolutionary history of strong traits conservatism (for example, strong environmental filtering), PD can be used as a good proxy for EF (the ancestral lineages). We would expect this situation to be reversed if the species that constitute a community at a particular time had been through different evolutionary histories (in our case the evolved lineages) or if they had experienced strong interspecific competition during trait differentiation [4] . This line of reasoning therefore requires gathering information not only just about the traits that are important for EF, but also whether they are conserved within the phylogeny. The next generation of experiments should assemble species belonging to different species pools with different evolutionary histories and degrees of traits conservatism to explore intermediate scenarios, and to discover the degree to which these results can be generalized. Ecologists have been preoccupied with the mechanisms underlying the relationship between species richness and EF [2] , [22] , in part because of the implications for conservation [3] , [23] . Such studies have focused on whether EF increases with the number of species because of functional complementary (for example, they feed on different resources), or because of the selection/sampling effect ( sensu ref. 22 ). PD has been proposed as useful to approximate functional diversity and thus EF under conditions where complementarity is important [14] , [16] . Our study proposes that 'phylogenetic selection effects' might also promote a positive phylogenetic–EF relationship. We found that ancestral lineages from one clade were more productive, and so the productivity of ancestral assemblages largely reflected whether a lineage from that clade was present. We also found that transgressive overyielding was rare implying that a selection effect dominates the positive PD–EF relationship. In that case, the amount of variance explained by PD was much greater than the variance explained by lineage diversity. Although there was relatively little evidence for transgressive overyielding overall, we found that the overyielding index did increase with PD of ancestral lineages for high lineage diversity treatments. This result suggests that the phylogenetic selection effect was weaker at high lineage diversity among these lineages. These lineage-rich communities are indeed more likely to contain at least one of the lineages from the highly productive clade, opening the possibility for complementarity to occur. Our results both emphasize the importance of using the community phylogenetic structure to predict EF as previously proposed [14] , [16] and warn against using this information without a good knowledge on past evolutionary history. Even if there are inherent limitations in using organisms with short generation times, experimental evolution provides an excellent method for disentangling the role of PD on EF. We have mainly illustrated that PD can provide information about EF when there is a strong conservatism of the traits important to EF. The importance of this signal will depend on the evolutionary history and environmental constraints experienced by co-occurring species and on the evolutionary lability of the traits providing EF. Effort will be now needed to explore the extent to which the traits that are the most associated to EF and species persistence within ecological communities are conserved within the phylogeny. We expect that evolution and genetics will strongly contribute to a full understanding of the biodiversity–EF relationship, and that future advances in this field will incorporate mechanisms of species adaptation and macroevolution [6] , [24] , [25] . Bacterial collection and experimental evolution We isolated 31 bacterial lineages from coastal seawater sampled off the Bay of Blanes, Spain (40°40′N-2°50′E) on two occasions on 20–21 February 2007 and 20–21 September 2007. Cell and colony morphotype descriptions were assessed and confirmed at each generation step. The 16S rDNA genes of the ancestral lineages were sequenced to construct the phylogenetic tree and to perform basic local alignment search tool analysis to infer their taxonomy. Likewise in most oceanic samples cultured on marine broth [26] , the isolates belong to the gamma-subclass of Proteobacteria, with a predominance of Psychrobacter species in the samples from February, which was expected because of low water temperature (~5 °C). Each lineage was individually submitted to a selection period on different single-carbon substrates of a BIOLOG Ecoplate (with three replicate lines per treatment). The microplates contain 31 different carbon sources (plus one blank) belonging to different chemical families. Each of the 31 strains was allocated at random to 1 of the 31 carbon substrates. We transferred the lineage to a fresh media every 48 h during 64 days of incubation at 20 °C. We conducted assays at the end of the selection period for each ancestral and evolved lineage (three replicates per strain) to measure individual strain performances on each carbon substrate at the end of the experiment. We incubated every strain on the 31 carbon substrates for 48 h at 20 °C. The Ecoplates were prepared with 120 μl of the buffered M9 solution. The Ecoplates were incubated with 30 μl of culture. Each strain/lineage was incubated in triplicate at 20 °C in humid chambers. Light absorbance at 590 nm was measured after 48 h. If the experimental manipulation had resulted only in physiological changes (for example, gene expression), the metabolic profiles (which substrates they metabolized) of each strain should converge, but this was not the case. The experimental selection resulted in a small but significant improvement in the overall ability of each lineage to exploit carbon sources (from an average of 3.9 carbon sources to 4.4, see ref. 13 ). Although the ancestral lineages were using only a subset of the different carbon substrates, the evolved lineages exploited a wider range of carbon substrates. After the isolation of the ancestors and the 30-s transfer, the content of every well was amended with glycerol (50% v/v) and frozen at −80 °C. The sequence data have been deposited in the GenBank Nucleotide database under accession codes HM246259 , HM246274 , HM246277 , HM246356 , HM246357 , HM246363 , HM246364 , HM246366 , HM246367 , HM246375 , HM246380 , HM246386 , HM246388 , HM246389 and HM246397 . Biodiversity and EF experiment We conducted a biodiversity-functioning experiment with lineage and PD as independent treatments, for both the ancestral and the evolved lineages. We subsampled randomly 16 lineages out of the 31 lineages that were isolated. Lineage diversity treatments were 1, 2, 4 and 8 lineages (from a pool of 16 lineages). For each lineage diversity treatment of 2, 4 and 8 lineages, we created 60 random assemblages with a gradient of PD (total of 180 assemblages + the monocultures). To do so, we first generated 1,000 random assemblages by sampling lineages without replacement from the 16 lineages and calculated the PD. Note that the distribution of PD tends to bimodality because of the shape of the phylogenetic tree. Low PD mixtures are found when the random sampling is conducted within a clade, and high diversity mixtures are found when it is conducted across clades. We randomly sampled a subset of 60 assemblages with a sampling probability inversely proportional to the frequency of the corresponding PD, which yields a uniform distribution of phylogenetic diversities. PD was calculated as the total phylogenetic branch length of the lineage present in the community [27] divided by the number of lineages present in the assemblage. Dividing by the number of lineages present in the assemblage results in comparable ranges of PD between lineage diversity treatments. Each assemblage was replicated three times. Each lineage was initially grown for 24 h at 20 °C in 5 ml of MB (a complex media made of yeast extracts, bacto peptone and salts; Beckson and Dickinson Difco Marine broth 2216; autoclaved for 20 min at 121 °C) media under constant orbital shaking in humid chambers. The cultures were then centrifuged (5 min at 3,500 r.p.m) and washed by removing the MB and adding 5 ml of M9 minimal salts (NH 4 Cl, 0.1 g l −1 ; Na 2 HPO 4 , 6 g l −1 ; KH 2 PO 4 , 3 g l −1 ; NaCl, 0.5 g l −1 ) with buffered salinity at 35.6 by the addition of NaCl to match salinity of the environment from which they were sampled. As the strains had different productivities in the MB, we first measured cell density by staining with Sybrgreen and measuring green fluorescence on a multiwell plate reader (FLUOstar OPTIMA spectrophotometer, BMG). Before constructing the assemblages, we adjusted the cell density to the concentration of the lineage with the lowest fluorescence measurement. The cultures were diluted 10 times with buffered M9 to obtain cell densities between 10 6 and 10 7 cells per ml. Bacterial lineages were then assembled in eight sterile 96 well–1 ml microplates. The bacteria were left in starvation for 2 h before 20 μl (40 μl for the monocultures) of each lineage was inoculated into the appropriate wells. Once the lineages were added to the appropriate wells of the eight plates, 10 μl of each assemblage was transferred into three replicated microplates (96 well–240 μl microplates) containing 140 μl of MB, for a total of 24 microplates. The cultures were incubated at 20 °C in humid chambers and productivity was approximated by measuring light absorbance at 660 nm after 48 h (FLUOstar OPTIMA spectrophotometer, BMG). Shown data are corrected by measured optical density of the blanks. Statistical analyses We tested the effect of PD and of lineage diversity on bacterial productivity by ANCOVA. Lineage diversity was treated as a categorical factor and PD as a continuous variable. The ANCOVA was performed independently for ancestral and evolved lineages. We then investigated whether the biodiversity–EF was the result of complementarity or selection effect. Under strong selection effects, we should expect the most productive species to dominate EF [28] . Transgressive overyielding occurs when the productivity in mixtures is greater than the productivity of the most productive species in the assemblage [22] . We thus considered that for a given assemblage, the expected productivity with only a selection effect should correspond to the productivity of the most productive species in the assemblage. The comparison between this expectation and the observed productivity allows us to approximate overyielding. We defined the overyielding index as log( Φ Mixture / Φ Max ) where Φ Mixture is the overall productivity of a given assemblage, and Φ Max is the maximum of the monoculture productivities of the lineages that are present in the assemblage [22] . We tested the effect of phylogenetic and species diversity on the overyielding index with the same ANCOVA model as for productivity. We tested the conservatism of productivity in monoculture and of functional similarity using Mantel tests. Functional similarity between species pairs was defined as the fraction of the 31 carbon substrates with the same usage (binary information, where 1 indicates a lineage is able to use the substrate). A lineage was considered able to use a given substrate when the optical density was larger than the 95% quantile of the blanks. Accession codes: The sequence data have been deposited in the GenBank Nucleotide database under accession codes HM246259 , HM246274 , HM246277 , HM246356 , HM246357 , HM246363 , HM246364 , HM246366 , HM246367 , HM246375 , HM246380 , HM246386 , HM246388 , HM246389 and HM246397 . How to cite this article: Gravel, D. et al . Phylogenetic constraints on ecosystem functioning. Nat. Commun. 3:1117 doi: 10.1038/ncomms2123 (2012).